Chimpanzees and humans harbour compositionally similar gut enterotypes Microbes inhabiting the human gastrointestinal tract tend to adopt one of three characteristic community structures, called ‘enterotypes’, each of which is overrepresented by a distinct set of bacterial genera. Here we report that the gut microbiotae of chimpanzees also assort into enterotypes and that these chimpanzee enterotypes are compositionally analogous to those of humans. Through the analysis of longitudinal samples, we show that the microbial signatures of the enterotypes are stable over time, but that individual hosts switch between enterotypes over periods longer than a year. These results support the hypothesis that enterotypic variation was present in populations of great apes before the divergence of humans and chimpanzees. The gut microbial communities in contemporary populations of humans have been partitioned into three clusters, termed ‘enterotypes’, each of which is characterized by a distinct set of overrepresented bacterial genera [1] . Whereas initially no relationship was detected between enterotypes and specific features of the host (such as age, health status, body morphotype, provenance or gender), recent work has revealed associations between enterotype and long-term diet: the Bacteroides -dominant enterotype is prevalent in individuals whose diets are high in animal fat and protein, whereas the Prevotella -dominant enterotype prevails in individuals with high-carbohydrate diets [2] . The assignment of the human gut microbiotae into discrete enterotypes raises several questions about the origins and evolution of these compositionally distinct microbial communities. If the formation of enterotypes is driven by the varied diets of human hosts [3] , enterotypes could have arisen in the human lineage over relatively recent timescales. But if enterotypes are the product of more ancient features, such as host immune system or gut physiology, they are likely to have originated before or during the diversification of the great ape species. Characterization of the gut microbial communities within populations of non-human great apes provides insights into the origins of the human enterotypes. Given the co-diversification between gut microbiotae and their great ape hosts [4] , [5] , [6] , [7] , the presence of compositionally similar enterotypes in humans and other great ape species, despite their present-day differences in diets and geographic distributions, would be consistent with the origination of enterotypes before the divergence of the human lineage. Here, we show that the gut microbiotae of chimpanzees assort into enterotypes that are compositionally analogous to those in humans, supporting the hypothesis that enterotypic variation was present before the divergence of humans and chimpanzees. Furthermore, through analyses of longitudinal samples, we show that the microbial signatures of chimpanzee enterotypes are stable over time, but that individual hosts shift among enterotypes over periods >1 year. Detection of enterotypes in chimpanzees To test for the presence of enterotypes in a non-human ape, we investigated the gut microbial communities within chimpanzees. One potential issue when comparing microbiotae across chimpanzees and humans is the large difference in levels of intraspecific genetic variation between the two groups: chimpanzees classify into multiple subspecies that diversified over the last 1.5 million years [8] , [9] , [10] , whereas the ancestry of all modern humans can be traced to population bottlenecks that occurred over the last 200,000 years [11] . Therefore, we restricted our analyses to the gut microbial communities within a single subspecies of chimpanzees ( Pan troglodytes schweinfurthii ), a monophyletic clade of approximately the same age as modern humans [10] . We tested for the presence of enterotypes in the gut microbiomes of 35 chimpanzees from the Gombe Stream National Park by using the same clustering and cluster validation methods that Arumugam et al. [1] utilized to identify the human enterotypes. These anaylses revealed that the chimpanzee microbiotae assort based on their genus-level compositions into three distinct clusters (that is, enterotypes) that do not significantly associate with host age, genealogy or gender ( Fig. 1a ). The bacterial taxa identified by between class analysis as contributing most significantly to each cluster were Faecalibacterium in chimpanzee enterotype 1, Lachnospiraceae in chimpanzee enterotype 2 and Bulleidia in chimpanzee enterotype 3 ( Fig. 1b ). 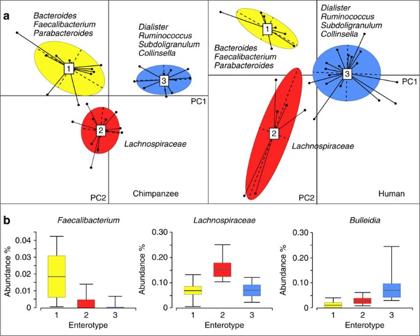Figure 1: Identification of chimpanzee enterotypes. (a) Assortment of gut microbial communities into enterotypes in chimpanzees and humans. Shown are BCA visualizations of enterotypes (coloured ellipses), as identified by PAM clustering, with black dots representing abundance distributions of bacterial genera from an individual host and numbered white rectangles marking the centre of each enterotype. Panel (right) showing human gut enterotypes modifed from Arumugamet al.1Bacterial taxa uniquely overrepresented in the corresponding chimpanzee and human enterotypes are listed. (b) Relative abundances of the three bacterial taxa that are principally responsible for the separation of chimpanzee enterotypes. Shown are means, ranges and first and third quartiles. Colour coding of enterotypes follows that in (a). Figure 1: Identification of chimpanzee enterotypes. ( a ) Assortment of gut microbial communities into enterotypes in chimpanzees and humans. Shown are BCA visualizations of enterotypes (coloured ellipses), as identified by PAM clustering, with black dots representing abundance distributions of bacterial genera from an individual host and numbered white rectangles marking the centre of each enterotype. Panel (right) showing human gut enterotypes modifed from Arumugam et al. [1] Bacterial taxa uniquely overrepresented in the corresponding chimpanzee and human enterotypes are listed. ( b ) Relative abundances of the three bacterial taxa that are principally responsible for the separation of chimpanzee enterotypes. Shown are means, ranges and first and third quartiles. Colour coding of enterotypes follows that in ( a ). Full size image Correspondence between human and chimpanzee enterotypes Although the gut microbial communities of the chimpanzees examined are compositionally more similar to one another than they are to the gut microbial communities of humans ( P =1.029 × 10 −86 , one-tailed t -test; Supplementary Fig. S1 ), all eight of the bacterial genera that are uniquely overrepresented in both a human and a chimpanzee enterotype show the same abundance patterns across enterotypes in both host species. Both human enterotype 1 and chimpanzee enterotype 1 are overrepresented by Bacteroides, Faecalibacterium and Parabacteroides ; human and chimpanzee enterotype 2 are overrepresented in Lachnospiraceae ; and human and chimpanzee enterotype 3 are overrepresented by Dialester, Ruminococcus, Subdoligranulum and Collinsella ( Fig. 1a ). There is broad correspondence between the chimpanzee and human enterotypes; however, several bacterial genera that are overrepresented in a chimpanzee enterotype are not overrepresented in any of the human enterotypes. For example, Anaerotruncus and Acetivibrio are overrepresented in chimpanzee enterotype 1, Anaerovibrio and Bifidobacterium are overrepresented in chimpanzee enterotype 2 and Bulleidia , Butyrivibrio , Coriobacteriaceae and Olsenella are overrepresented in chimpanzee enterotype 3, but these genera are either absent from or do not significantly contribute to the human enterotypes ( Table 1 ). Table 1 Frequencies of bacterial taxa uniquely overrepresented within each chimpanzee enterotype. Full size table Similarly, several bacterial genera that contribute to a human enterotype are not overrepresented in any of the chimpanzee enterotypes. The most prominent of these is Prevotella , which predominates in human enterotype 2, but is recovered at very high frequencies in all three chimpanzee enterotypes, accounting for 7.3% of chimpanzee enterotype 1, 8.4% of chimpanzee enterotype 2 and 9.9% of chimpanzee enterotype 3. Temporal and compositional stability of enterotypes The human enterotypes were identified initially from individual samples from a broad spectrum of hosts, a sampling scheme that does not allow examination of the temporal stability of enterotypes within hosts. For seven of the chimpanzees the gut microbial communities were assessed at multiple time points over an 8-year period ( Fig. 2 ). In all of these chimpanzees, there was a change in enterotype assignment during the 8-year sampling period, with three chimpanzees showing the identical configuration, harbouring enterotype 1 in years 2000 and 2001, and enterotype 3 in 2008. Despite the replacement of enterotypes within hosts, the compositional profiles of the enterotypes are robust to the inclusion of samples from different time points, with the primary bacterial drivers of enterotypes remaining constant for each iteration of partitioning around medoids (PAM) clustering. 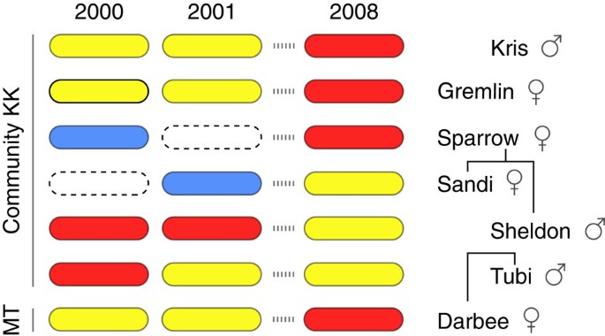Figure 2: Chimpanzee enterotypes vary within individuals over time. Enterotype assignments in individual chimpanzee hosts sampled longitudinally in 2000, 2001 and 2008. Samples assigned to enterotype 1 are represented by yellow capsules, samples assigned to enterotype 2 are represented by blue capsules, samples assigned to enterotype 3 are represented by red capsules and empty capsules indicate years when samples for a particular host were not analysed. Hosts are arranged by Gombe community affiliation (MT or KK), with gender and genealogy indicated (such that Sparrow is the mother of Sandi and Sheldon, and Tubi and Darbee are siblings). Figure 2: Chimpanzee enterotypes vary within individuals over time. Enterotype assignments in individual chimpanzee hosts sampled longitudinally in 2000, 2001 and 2008. Samples assigned to enterotype 1 are represented by yellow capsules, samples assigned to enterotype 2 are represented by blue capsules, samples assigned to enterotype 3 are represented by red capsules and empty capsules indicate years when samples for a particular host were not analysed. Hosts are arranged by Gombe community affiliation (MT or KK), with gender and genealogy indicated (such that Sparrow is the mother of Sandi and Sheldon, and Tubi and Darbee are siblings). Full size image The communities of microbes infecting the guts of chimpanzees ( P. t. schweinfurthii ) from the Gombe National Park assort into three compositionally distinct enterotypes that parallel those that have been recognized in human populations. All of the bacterial genera that are overrepresented in both the human and the chimpanzee enterotypes show the same compositional patterns in both host species. For example, both human enterotype 1 and chimpanzee enterotype 1 are enriched in Bacteroides, Faecalibacterium and Parabacteroides, whereas human and chimpanzee enterotype 2 are both overrepresented in Lachnospiraceae . Despite the overall congruence between the human and chimpanzee enterotypes, there are differences between host species in the prevalence of several bacterial genera ( Table 1 ), most notably in the distribution of Prevotella . Human enterotype 2 is distinguishable from the other human enterotypes by being enriched in Lachnospiraceae (as in chimpanzees) but also in its overrepresentation of Prevotella. In contrast, there are equally high frequencies of Prevotellae in each of the chimpanzee enterotypes. In humans, the Prevotella- dominant enterotype is associated with high-carbohydrate diets [2] , such that the consistently high level of Prevotella in chimpanzees is consistent with a typical chimpanzee diet, which is dominated by carbohydrate-rich fruits. That enterotypes are present both in humans and in chimpanzees suggests that enterotypic variation is an ancestral feature of the great ape microbiota. The compositional relatedness between the human and chimpanzee enterotypes is consistent with the origination of enterotypes before the human–chimpanzee split and the subsequent co-divergence between enterotypes and their hosts. Although the dissemination of bacterial taxa among host species could potentially generate similarities between human and chimpanzee enterotypes, such transfers cannot fully explain the presence of bacterial taxa that distinguish enterotypes in only one of the host species ( Tables 1 , 2 ). Detection of compositionally divergent enterotypes in other primates would further support the existence of enterotypes during great ape diversification; however, there is currently not sufficient sampling to characterize the intraspecific variation in microbiota composition outside the Hominini . In addition, several bacterial genera were detected in only a single host species ( Table 3 ). Nearly, 5% of the human faecal flora is comprised of these bacterial genera, some of which have been implicated in gastrointestinal tract diseases. For example, the mucin-degrading Akkermansiae have been linked to colitis [12] , Eggerthellae are enriched in patients with Crohn’s disease [13] and Coprobacilli are associated with certain forms of irritable bowel syndrome [14] . Table 2 Bacterial taxa predominating within each chimpanzee enterotype. Full size table Table 3 Frequencies of bacterial genera recovered only from humans or from chimpanzees. Full size table A standing question about human enterotypes is whether or not they are variable within an individual over time [1] , [2] . We have addressed this question in chimpanzees by assessing the variability of enterotype assignment within chimpanzee hosts sampled over an 8-year period. In short, each of the chimpanzee hosts that were assayed at multiple time points changed enterotypes over the sampling period ( Fig. 2 ). As observed in humans, there is no obvious association between chimpanzee enterotype and host genetics or geography. When sampled in 2000, the siblings, Sandi and Shelton, and their mother, Sparrow, each possessed different enterotypes, and their enterotypes changed, and still differed, in later samplings. Meanwhile, three chimpanzees that are not all members of the same family or same geographic community (Darbee, Gremlin and Kris) harboured the same enterotypes at each of the three time points sampled. In humans, diet is likely to be a major contributor to a host’s enterotype [2] . As the availability of different foodstuffs in Gombe can fluctuate seasonally [15] , [16] , diet may also influence the possession of certain chimpanzee enterotypes. However, we found no consistent association between enterotype and the season in which a host was sampled. Furthermore, all three enterotypes were present during each wet season when foods were abundant and the diets among the chimpanzee hosts were the most homogenous. That the same chimpanzee enterotypes were repeatedly recovered over the course of 8 years of sampling demonstrates that enterotypes reflect ecological communities that are reproducible both within and among hosts. But because enterotypes represent divisions within a continuous character (that is, the relative frequencies of numerous bacterial taxa within hosts), hosts that have the same enterotype need not have identical microbial communities. This variation can obscure the divisions between enterotypes: for example, Wu et al. [2] suggest that humans can be classified into two, not three, enterotypes, and we found support for both two and three chimpanzee enterotypes in this study ( Supplementary Figs S2 and 3 ). In sum, we have shown that chimpanzees possess enterotypes that are compositionally similar to those observed within human populations. Although the compositions of enterotypes remain stable, the particular enterotype harboured by an individual host can changes over the course of a year. We consider the enterotypic changes observed in chimpanzees as indications that human enterotypes are likely to shift several times over the lifespan of a host. Sample sources Genus-level abundance distributions of bacteria present in the guts of 33 humans from diverse geographic regions (Italy, France, Japan and USA) were retrieved from Arumugam et al. [1] , as provided by Dr. Peer Bork (EMBL Biocomputing, Heidelberg, Germany). Species-level abundance distributions for bacteria present in the guts of 35 chimpanzees ( P. t. schweinfurthii ) from the Gombe National Park were retrieved from Degnan et al. [1] and converted into genus-level distributions to enable direct comparisons between the human and chimpanzee data sets. We decided to focus our analyses on the single chimpanzee subspecies P. t. schweinfurthii , a monophyletic clade of approximately the same age as humans [8] , [9] , [10] , [11] , to avoid the confounding effects of excessive genetic variation among hosts. Clustering abundance distributions We applied methods described by Arumugam et al. [1] to test for the presence of enterotypes in chimpanzees and to compare enterotypes across humans and chimpanzees. We applied PAM clustering to the genus-level relative abundance profiles of chimpanzees and humans, setting the number of clusters a priori from two to ten and using the same probability distribution distance metric (that is, the square root of the Jensen–Shannon divergence) implemented by Arumugam et al. [1] Ordination of human and chimpanzee microbiotae To evaluate whether chimpanzees and humans possess compositionally distinct microbiomes, we calculated pairwise Bray–Curtis dissimilarities of genus-level abundance distributions between samples in QIIME version 1.4.0 (ref. 17 ). Pairwise dissimilarities were statistically evaluated with one-tailed t -tests and visualized by principal coordinates analysis ( Supplementary Fig. S1 ). Enumeration of enterotypes To determine the optimal number of clusters (that is, enterotypes) in each data set, the Calinski–Harabasz (CH) index and the silhouette score were calculated for each set of clusters generated by PAM clustering. We chose for subsequent analyses the number of clusters that maximized the CH index for each data set ( Supplementary Fig. S2 ). The CH index for a set of clusters is proportional to the ratio of the between-cluster sum-of-squares to the within-clusters sum-of-squares, with higher CH values indicating a better fit between the clustering and the data [18] . Silhouette scores were also calculated for each set of clusters but failed to differentiate between two and three clusters ( Supplementary Fig. S3 ). Bacterial contributors to enterotypes Between-class analysis (BCA) was implemented as in Arumugam et al . [1] using the ade4 package in R to identify the bacterial genera most responsible for the observed clustering in the chimpanzee data set. BCA is a form of principal component analysis with respect to an instrumental variable [19] , which, in this case, is the cluster/enterotype assignment of each abundance distribution. Only genera with an average abundance >0.01% across samples were considered. Detection of overrepresented genera We used Fisher’s exact test to identify overrepresented genera in each of the chimpanzee enterotypes. As in Arumugam et al. [1] , we adopted a conservative approach by considering only those genera that were overrepresented in a single cluster. Correction for multiple testing was based on the Benjamini–Hochberg false discovery rate, with the corrected P -value cutoff set at 0.05. Detection of bacterial genera specific to a host species Arumugam et al. [1] generated taxonomic assignments for the sanger metagenome data set by assigning reads to a database of 1,511 bacterial genomes, whereas Degnan et al. [1] generated taxonomic assignments for the 16s rRNA data set by assigning reads to the RDP database, which contains a greater breadth of bacterial taxa than the database used by Arumugam et al. [1] To circumvent potentially confounding effects that this discrepancy in taxonomy assignment may have on the identification of bacterial genera unique to each host species, we retrieved the 16s rRNA data set of Turnbaugh et al. [20] and assigned taxonomy following the methods of Degnan et al. [1] We then identified bacterial genera unique to each host species by comparing the taxonomic assignments of Degnan et al. [1] with those of Arumugam et al. [1] as well as those produced from Turnbaugh et al. Testing for the stability of enterotypes The longitudinal samples from seven chimpanzees reported in Degnan et al. [1] were used to evaluate the temporal stability of gut enterotypes. We detected enterotypic changes via two approaches. First, we established the enterotype for each host in the most recent (that is, 2008) sample for each individual and then repeated the analysis after substituting a single sample from an earlier time point (2000 or 2001), such that only one abundance distribution differed between any two iterations of the PAM clustering. Second, we clustered all samples from all individuals simultaneously in one iteration of PAM clustering. The two approaches for detecting enterotypic change produced identical results ( Fig. 2 ). How to cite this article: Moeller, A. H. et al. Chimpanzees and humans harbour compositionally similar gut enterotypes. Nat. Commun. 3:1179 doi: 10.1038/ncomms2159 (2012).